High-efficiency Cooper pair splitting demonstrated by two-particle conductance resonance and positive noise cross-correlation Entanglement is at the heart of the Einstein-Podolsky-Rosen paradox, where the non-locality is a necessary ingredient. Cooper pairs in superconductors can be split adiabatically, thus forming entangled electrons. Here, we fabricate such an electron splitter by contacting an aluminium superconductor strip at the centre of a suspended InAs nanowire. The nanowire is terminated at both ends with two normal metallic drains. Dividing each half of the nanowire by a gate-induced Coulomb blockaded quantum dot strongly impeds the flow of Cooper pairs due to the large charging energy, while still permitting passage of single electrons. We provide conclusive evidence of extremely high efficiency Cooper pair splitting via observing positive two-particle correlations of the conductance and the shot noise of the split electrons in the two opposite drains of the nanowire. Moreover, the actual charge of the injected quasiparticles is verified by shot noise measurements. Two particles are entangled if a detection or a manipulation of the quantum state instantaneously affects the other quantum state. Hence, being non-local, the entanglement of two separated particles must involve simultaneous, non-local, measurements. Such two-particle state can be achieved, in principle, via particles interaction or by breaking apart a composite quantum object. For example, fully entangled photons are readily provided by low-efficiency parametric down-conversion of higher energy photons [1] , [2] , [3] . Such a feat is not readily available for electrons. However, the closest electrical analogue to the high energy photons are Cooper pairs in a superconductor, being a natural source of entangled electron pairs. Splitting them adiabatically may give birth to entangled electron pairs. Indeed, it had been predicted and measured that Cooper pairs, emanating from a superconductor, can split into two normal metallic leads in the so-called cross Andreev reflection process [4] , [5] , [6] , [7] , [8] , [9] , [10] , [11] . Such process can be conclusively verified by observing positive coincident arrival events, namely, positive cross-correlation of current fluctuations in two separated normal metallic leads that collect the split pairs [12] , [13] , [14] , [15] , [16] , [17] , [18] . The main difficulty in identifying such process is the overwhelming flux of Cooper pairs that enters the normal leads via direct Andreev reflection (the proximity effect). Such an experiment was attempted by Wei et al . [10] , where cross-correlation measurements were performed in an all metallic system (Al superconductor and Cu normal metal) without quantum dots (QDs) at very low frequencies (2–6 Hz) at a temperature of 0.3–0.4 K. The large 1/ f noise, the relatively high temperature and a dominant Cooper pair transport compromised the obtained data. Replacing each of the normal metallic leads with a QD in the Coulomb blockade regime (see ref. 12 ), performed by Hofstetter et al. [8] , indeed suppressed Cooper pairs transport, but lacked to prove coincidence splitting. Here, we provide results of coincidence measurements by observation of positive cross-correlation of current fluctuations. These are reinforced by simultaneous non-local conductance measurements on both sides of the nanowire. Quenching superconductivity with a weak magnetic field suppressed the positive correlations. We obtained a splitting efficiency, defined as the ratio between single-electron to two-electron transport, as high as ~100%. 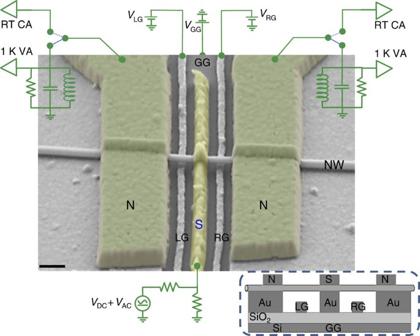Figure 1: Device and measurement setup. An SEM image, with false colour enhancement, of the working suspended InAs-based splitting device. Scale bar, 200 nm. The nanowire is connected in its centre with a superconducting Al contact (S) and two normal Au contacts (N) each on either sides of the nanowire. Inset shows a cross-sectional schematic view. The superconducting contact is biased by a voltage source and the currents at the two normal drains are measured by room temperature current amplifiers (RT CA). Current fluctuations are measured by cold voltage amplifiers (1 K VA) with an inductance-capacitance (LC) resonant circuits at their input. The switching between RT CA and 1 K VA is done by a low-temperature relay. Experimental setup Figure 1 shows a SEM image of our device, as well as a schematic illustration of the measurement setup. A 50-nm diameter InAs nanowire, grown by a high purity Au-assisted MBE process [19] , was suspended on Au pillars above a conducting Si substrate coated with 150 nm SiO 2 . A superconducting aluminium strip (S), ~100 nm wide, was intimately contacted at the centre of the nanowire, separating it into two equal sections, each ~200 nm long, with two terminating gold ohmic contacts serving as drains (D). Aside from the conducting Si substrate, which served as a global gate (GG), two narrow metallic gates, some 50 nm wide, were used to tune the local chemical potential on each side of the nanowire. Although the local gates (positively biased) accumulated electron puddles, the GG (negatively biased) induced barriers on the sides of each puddle, thus forming two QDs on both sides of the superconducting contact. Although currents were amplified with a room temperature current amplifier at ~575 Hz, current fluctuations (broad band auto-correlation or shot noise) and their cross-correlation, were first filtered by an inductor-capacitor (LC) resonant circuit tuned to 725 kHz (bandwidth ~100 kHz); amplified by a home-made cold (1 K) preamplifier cascaded by a room temperature amplifier, and finally measured by a spectrum analyser or an analogue cross-correlation setup. More details of the fabrication process and the measurement techniques are given in the Methods section. Figure 1: Device and measurement setup. An SEM image, with false colour enhancement, of the working suspended InAs-based splitting device. Scale bar, 200 nm. The nanowire is connected in its centre with a superconducting Al contact (S) and two normal Au contacts (N) each on either sides of the nanowire. Inset shows a cross-sectional schematic view. The superconducting contact is biased by a voltage source and the currents at the two normal drains are measured by room temperature current amplifiers (RT CA). Current fluctuations are measured by cold voltage amplifiers (1 K VA) with an inductance-capacitance (LC) resonant circuits at their input. The switching between RT CA and 1 K VA is done by a low-temperature relay. Full size image One side transport and charge measurement With all three gates unbiased, the InAs nanowire conductance is n-type with an approximate electron density of 5 × 10 6 cm −1 . The differential conductance of one side of the wire, say the left side, when the right side is pinched-off by its local gate (RG), is measured at 10 mK as a function of its gate voltage ( V LG ), whereas the GG is grounded. The conductance varies around 2 e 2 / h ( Fig. 2a )—characteristic of Fabry-Perot type oscillations [19] . Note that conductance exceeding 2 e 2 / h for the first subband indicates the presence of Andreev reflections with a barrier near the S–InAs interface (with maximum of 4 e 2 / h ). Under similar conditions, the non-linear differential conductance as a function of bias V SD is shown in Fig. 2b for two values of V LG (C and A in Fig. 2a ). The gate voltage V LG mainly controls the barrier near the S–InAs interface, shifting the linear conductance from high at point C to low at point A, with a strikingly different non-linear conductance in the two points. At point C, with a linear transmission probability t * =2.6/4=0.65, the conductance drops with bias—as expected for a diminishing tunnelling probability of Cooper pairs as the bias approaches half the superconducting gap (Δ). Alternatively, at point A, with t * =0.4, the conductance increases with bias and peaks at V SD =Δ. Here single electron tunnelling dominates. The superconducting gap 2Δ ~220 μeV is noted by the dotted line. 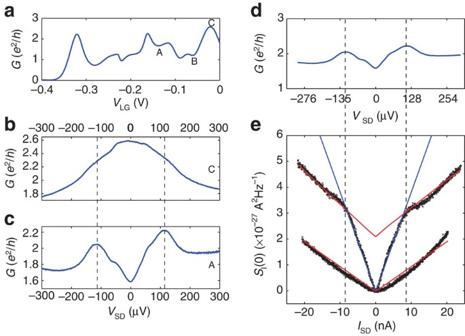Figure 2: Andreev reflection and charge measurement. (a) Differential conductance (G) of the left side of the nanowire as a function of left local gate voltage (VLG) when the right side is pinched off. (b,c) Bias (VSD)-dependent differential conductance at points C and A, respectively. In C, the conductance is characteristic of Andreev reflection in a superconductor–normal (S–N) junction. In A, it is characteristic of a tunnelling in a superconductor–insulator–normal (S–I–N) junction. Dashed lines border the superconducting gap (2Δ). (d) Non-linear conductance and (e) auto correlation signal (shot noise) as a function of current (ISD) for magnetic fields,B=0 andB=0.2 T. Solid lines are theoretical predictions at temperature,T=10 mK. Charge is 2eforVSD<Δ (blue line) andeforVSD>Δ (red line). A perpendicular magnetic field quenches the non-linear differential conductance with a critical field B ~0.12 T. Figure 2: Andreev reflection and charge measurement. ( a ) Differential conductance ( G ) of the left side of the nanowire as a function of left local gate voltage ( V LG ) when the right side is pinched off. ( b , c ) Bias ( V SD )-dependent differential conductance at points C and A, respectively. In C, the conductance is characteristic of Andreev reflection in a superconductor–normal (S–N) junction. In A, it is characteristic of a tunnelling in a superconductor–insulator–normal (S–I–N) junction. Dashed lines border the superconducting gap (2Δ). ( d ) Non-linear conductance and ( e ) auto correlation signal (shot noise) as a function of current ( I SD ) for magnetic fields, B =0 and B =0.2 T. Solid lines are theoretical predictions at temperature, T =10 mK. Charge is 2 e for V SD <Δ (blue line) and e for V SD >Δ (red line). Full size image For the above conditions, with the barrier at the S–InAs interface, the injected current is carrying shot noise, which depends linearly on the injected current ( I ) and the tunnelling charge ( e * ) [20] , [21] , [22] , [23] . The low frequency spectral density of the excess noise (shot noise above the Johnson-Nyquist and environment noise) in the single InAs channel takes the form: S i (0)=2 e * I (1− t * ) F ( T ), with t * = t for electrons and t * = t 2 for Cooper pairs, and F ( T )=cothζ−1/ζ, with ζ= e * V SD / k B T . Determination of the non-linear conductance ( Fig. 2b ) is crucial for accurate excess noise value as it affects the background noise (composed of thermal and current noise of the preamplifier [24] ); as explained further in the Supplementary Fig. S2 . In Fig. 2e , we plot S i (0) as a function of I for zero magnetic field B and for B ~0.2 T. The blue and red solid lines are the 10-mK predictions for t * =0.4, e * =2 e and t =0.63, e * = e , respectively; demonstrating an excellent quantitative agreement with the data (black circles). The distinct change of slope (from e * =2 e to e * = e ) nicely corresponds to Δ that was deduced from the conductance ( Fig. 2d ). A perpendicular small magnetic field (~0.2 T) quenched the superconductivity with the excess noise nicely agreeing with e * = e across the full biasing range. QD and Cooper pair splitting We now turn to study the efficiency of Cooper pair splitting. Introducing a Coulomb blockaded QD on each side of the nanowire is expected, under suitable conditions, to suppress Cooper pair transport due to the dot’s relatively large charging energy U . Preventing single electron injection from the superconductor necessitates, eV SD , k B T <Δ, while quenching of Cooper pairs transport through the QD requires eV SD < U . The characteristic energies of each QD is determined by measuring the non-linear differential conductance as a function of the DC bias ( V SD ) and the local gate voltage (via the so-called diamond structure; see Supplementary Fig. S3 ). We estimated the average charging energy at U =8–10 meV and the single particle level broadening at Γ ~200–300 μeV. Under these conditions, with U >Δ but Γ≈Δ> k B T , two-sequential-electron transport, proportional to (Γ/Δ) 2 , is barely suppressed [12] . The efficiency, defined as the ratio of splitted current/Cooper pair current, η= I e / I CP , can be expressed as with , where ξ is the coherence length of a Cooper pair, k F , the Fermi wave vector and δ r = r 1 − r 2 , the distance between the emerging split electrons; with all values related to the proximity region in the InAs [12] . As δ r is likely to be smaller than the superconductor width, we believe that its suppression factor is not important, leading to η (πΔ/Γ) 2 ~1. Non-local conductance measurements We begin with non-local conductance measurements by forming two QDs on both sides of the nanowire. Applying a large negative voltage to the GG ( V GG =−15 V), while keeping the local gates ( V LG and V RG ) at small negative voltage, induces two barriers surrounding each of the two electron puddles. Starting, with the left QD L , although the right side of the nanowire is blocked, the conductance peaks as a function of V LG are solely due to Cooper pairs transport. Such transport takes place likely due to sequential tunnelling of single particles by higher order process within a time scale smaller than the coherence time of a Cooper pair; leading to a finite conductance proportional to (Γ/Δ) 2 (ref. 12 ). Now when the right side of the nanowire is also allowed to conduct, Cooper pairs splitting can take place, thus also enhancing current on the left side. The largest one-electron transport on both sides is expected when the two QDs are at resonance ( Fig. 3a ), which is actually a two-particle conductance resonance [12] . Such non-local conductance measurement is shown in Fig. 3b . We simultaneously measure the conductance of both sides of the nanowire by two individual current amplifiers. In Fig. 3b colour plot of G L is plotted by scanning the V RG for different fixed values of V LG . The solid red line towards the left side of the colour plot as a function of V LG is the measured G L of one Coulomb blockade peak due to Cooper pairs transport through QD L when the right side is blocked, I CP . The blue line on the top panel is the local conductance of QD R as a function of V RG when the left side is blocked. Tunning to V LG =−0.558 V (the dashed white line in Fig. 3b ) and scanning V RG leads to the non-local G L (projected red line). Conductance is enhanced (Δ G , due to single electron transport, I e ) by as much as 0.18 e 2 / h (marked by a asterik in Fig. 3b ), corresponding to the conductance peaks of QD R with V RG . The efficiency of splitting, defined as η= I e / I CP =Δ G / G , is proportional to t R / t L for the left side. For tuning V LG =−0.558 V, the efficiency is ~70% (Δ G / G =0.18/0.26) and is more than 100% when V LG is set to off resonance (see Supplementary Fig. S4a ). 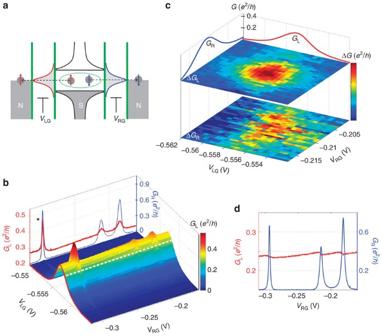Figure 3: Non-local conductance measurement. (a) Band diagram of the system aligned for maximum Cooper pair splitting. In the non-local measurement, we look at the conductance of one side of the nanowire (with an embedded QD) as a function of local gate voltage applied to the QD on the other side. (b) Colour plot of the left side conductanceGLby scanning the right local gate voltages,VRGfor different fixed values of left local gate voltages,VRG. The solid red line towards the left side of the colour plot is a Coulomb blockade peak of QDLdue to Cooper pairs transport when the right side is blocked. The projected red line on the top panel is the non-local conductanceGLmeasured as a function ofVRG(for the white dashed line atVLG=−0.558 V), with peaks enhanced in a corresponding manner to the conductance peaks of QDR(blue line on the top panel). (c) 2D colour plot of currents due to Cooper pair splitting through the left QD (ΔGL) and the right QD (ΔGR−scaled up by × 2). The red and blue lines at top left and top right panel are the Coulomb blockade peaks of QDLand QDRnearVLG=−0.557 V andVRG=−0.21 V, respectively. (d) Non-local signal ofGL(red line) as a function ofVRGforVLG=−0.558 V atB=0.2 T. The blue line is the localGRas a function ofVLG. Figure 3: Non-local conductance measurement. ( a ) Band diagram of the system aligned for maximum Cooper pair splitting. In the non-local measurement, we look at the conductance of one side of the nanowire (with an embedded QD) as a function of local gate voltage applied to the QD on the other side. ( b ) Colour plot of the left side conductance G L by scanning the right local gate voltages, V RG for different fixed values of left local gate voltages, V RG . The solid red line towards the left side of the colour plot is a Coulomb blockade peak of QD L due to Cooper pairs transport when the right side is blocked. The projected red line on the top panel is the non-local conductance G L measured as a function of V RG (for the white dashed line at V LG =−0.558 V), with peaks enhanced in a corresponding manner to the conductance peaks of QD R (blue line on the top panel). ( c ) 2D colour plot of currents due to Cooper pair splitting through the left QD (Δ G L ) and the right QD (Δ G R −scaled up by × 2). The red and blue lines at top left and top right panel are the Coulomb blockade peaks of QD L and QD R near V LG =−0.557 V and V RG =−0.21 V, respectively. ( d ) Non-local signal of G L (red line) as a function of V RG for V LG =−0.558 V at B =0.2 T. The blue line is the local G R as a function of V LG . Full size image Similarly, non-local enhancement of G R induced by V LG takes place (see Supplementary Fig. S4b ). A full representation of the non-local conductance, Cooper pair splitting currents, between the left QD (Coulomb blockade peak at V LG =−0.557 V) and the right QD (Coulomb blockade peak at V RG =−0.21 V) is shown in the two colour plots in Fig. 3c ; with Δ G L ( V LG , V RG ) (top representation) and Δ G R ( V LG , V RG ) (bottom representation). Note that the apparent Δ G L is bigger than Δ G R . The two-particle conductance resonance can be seen in Fig. 3c , where each single particle transport is non-local, as it depends on the transmission of both QDs ( t L t R ). Here, we have shown the resonance of split electrons with an energy close to the Fermi energy. In the presence of magnetic field (~0.2 T), the superconductivity quenches and the non-local conductance diminishes ( Fig. 3c ). The residual non-local conductance, in the form of a weak saw-tooth-like dependence, is the familiar detection behaviour of electron occupation in QDs [25] . Owing to the proximity between the two dots (~300 nm), the left dot senses the potential swing in the right dot when an electron is added to it, thus affecting its conductance. Cross-correlation measurements Measuring positive cross-correlation of current fluctuations in the two drains, assuring coincident clicks, provides direct test for the existence of split Cooper pairs (as the Andreev reflections on each side are uncorrelated). To measure the cross-correlation, the current fluctuations were first amplified by a home-made cooled preamp, with the amplified signals fed to an analogue signal multiplier at 725 kHz. Starting with an unbiased device, the uncorrelated background noise in both drains was nulled (being only some 2–3% of the actual auto-correlated back ground noise due to cross talk, see Supplementary Fig. S5 ). In Fig. 4a the cross-correlation, measured with the two dots around their respective resonances ( V LG =−0.557 V and V RG =−0.21 V), is displayed for V SD =20, 10 and 5 μV DC. The cross-correlation is positive and is highest when the two dots are at resonance; in full agreement with the nonlocal conductance measurement ( Fig. 3c ). The dependence of the cross-correlation signal on V SD , for the two QDs at resonance, is shown in Fig. 4c . Applying a perpendicular magnetic field, B =0.2 T, quenches the superconductivity and thus eliminates the (positive) correlation between the drains’ current fluctuations ( Fig. 4b ). 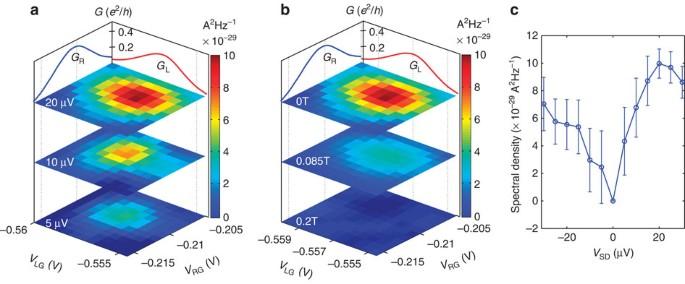Figure 4: Noise cross correlation. Cross-correlated noise measured by a cross-correlation setup. The current fluctuations from the normal contacts are filtered by two individual inductor-capacitor (LC) circuits with a matched resonant frequency of 725 kHz with the amplified signals (by cold amplifiers) fed into an analogue signal multiplier (at 725 kHz with a band width of 100 kHz). (a) Positive cross-correlation signals for bias voltages,VSD=20, 10 and 5 μV between left side (Coulomb blockade peak of the QDLat left local gate voltage,VLG=−0.557 V) and right side (Coulomb blockade peak of the QDRat right local gate voltage,VRG=−0.21 V). (b) Cross-correlation signal for magnetic fields,B=0, 0.085 and 0.2 T (VSDis kept at 20 μV). (c) Power spectral density of cross-correlation,SCCas a function ofVSD, measured when both dots are at resonance. Error bars are calculated from the standard deviations. Figure 4: Noise cross correlation. Cross-correlated noise measured by a cross-correlation setup. The current fluctuations from the normal contacts are filtered by two individual inductor-capacitor (LC) circuits with a matched resonant frequency of 725 kHz with the amplified signals (by cold amplifiers) fed into an analogue signal multiplier (at 725 kHz with a band width of 100 kHz). ( a ) Positive cross-correlation signals for bias voltages, V SD =20, 10 and 5 μV between left side (Coulomb blockade peak of the QD L at left local gate voltage, V LG =−0.557 V) and right side (Coulomb blockade peak of the QD R at right local gate voltage, V RG =−0.21 V). ( b ) Cross-correlation signal for magnetic fields, B =0, 0.085 and 0.2 T ( V SD is kept at 20 μV). ( c ) Power spectral density of cross-correlation, S CC as a function of V SD , measured when both dots are at resonance. Error bars are calculated from the standard deviations. Full size image According to our model, the non-local conductance is expected to be proportional to t L t R , and Δ G R =Δ G L . This was not observed. Although we do not understand the reason for this discrepancy, it might be related to a reduction in the two-electron transport, be it Cooper pairs or sequential two-electron transport, accompanying the single electron transport. Near the resonance of the QD, charge fluctuations and thus wide frequency range potential fluctuations are dominant and can partly dephase the neighbouring dot (see such saw-tooth behaviour in Fig. 3d ), possibly affecting the higher order two-electron transport. The spectral density of the cross-correlation signal at zero temperature is given by S CC =<Δ I L Δ I R > 2 eI CAR (1− t ), with I CAR the single electron current (due to cross-Andreev reflections) on one side [17] . As I CAR / I AR ~0.14 (0.04/0.3 seen in Fig. 3c for the resonance peaks near V LG =−0.557 V and V RG =−0.21 V) and I AR =500 pA at V SD =30 μV, I CAR =70 pA. Hence, we expect S CC ~1.7 × 10 −29 A 2 Hz −1 . However, the experimentally obtained S CC ~7–10 × 10 −29 A 2 Hz −1 is more than four times higher than the estimated value. This discrepancy may be attributed to an under-estimated value of Cooper pair splitting efficiency that is deduced from the non-local conductance measurement. In conclusion, we have shown Cooper pair splitting efficiency with ratio approaching unity of split pairs vs unsplit pairs by measuring average and time-dependent cross-correlations of two electron transport. To prove the entanglement, one still needs to show Bell's inequality by measuring the coherence and spin correlation using ferromagentic contacts. Device fabrication The sample was fabricated on a thermally oxidized Si. The nanowire was suspended on three gold pillars, ~50 nm high. Two lower gold pillars, ~25 nm high, provided local gating on both sides of the wire. After wires spreading from the ethanol solution, the source and drain regions were etched by ammonium polysulphide ((NH 4 ) 2 S x =1.5 M ) to remove the native oxide, and were immediately transferred into the evaporation chamber. For normal-metallic contacts 5/100 nm Ti/Au were evaporated, whereas for the superconducting contact 5/100 nm Ti/Al was used. Measurement technique The superconducting contact was biased by a voltage source, DC or AC (the voltage divider was placed on the cold finger, see Supplementary Fig. S1 ), with an AC excitation voltage of ~2 μV. Conductance measurements were conducted at a rather low frequency (room temperature current preamplifier at 575 Hz; gain 10 7 , input impedance ~200 ohm and current noise ), as well as at a higher frequency (cooled to 1 K voltage preamplifier at 725 kHz, gain 2.5, voltage noise and current noise ). At the input of the ‘cold’ preamplifier, a LCR circuit determined the frequency 725 kHz and the bandwidth (100 kHz). The amplified signal is fed to a room temperature ‘NF amplifier’, followed by a spectrum analyser with a bandwidth of 30 kHz. To switch between the two measurement systems a ‘Relay’, placed at the base temperature, was operated by a 100-ms, 1 V pulse. For cross-correlation measurements, we employed an analogue cross-correlation setup, where the signals from the two NF amplifiers were multiplied and measured by a digital multimeter (at a bandwidth of 100 kHz). How to cite this article: Das, A. et al. High-efficiency Cooper pair splitting demonstrated by two-particle conductance resonance and positive noise cross-correlation. Nat. Commun. 3:1165 doi: 10.1038/ncomms2169 (2012).